An upconverted photonic nonvolatile memory Conventional flash memory devices are voltage driven and found to be unsafe for confidential data storage. To ensure the security of the stored data, there is a strong demand for developing novel nonvolatile memory technology for data encryption. Here we show a photonic flash memory device, based on upconversion nanocrystals, which is light driven with a particular narrow width of wavelength in addition to voltage bias. With the help of near-infrared light, we successfully manipulate the multilevel data storage of the flash memory device. These upconverted photonic flash memory devices exhibit high ON/OFF ratio, long retention time and excellent rewritable characteristics. Infrared (IR) light is in the electromagnetic spectrum between the visible and microwave portions, and exhibits extensive applications in thermography, night vision, energy conversion, spectroscopy, medical and telecommunication [1] , [2] , [3] , [4] , [5] . Near-IR energy (750–1,000 nm) can also be further applied in implantable electronic devices since its long wavelength allows it to penetrate deep into tissues, and its low energy is not harmful to healthy cells [6] , [7] . In this regard, IR-based electronic devices are under vigorous studies in both academia and industry for the rapid development of portable and flexible electronics [8] , [9] . Nonvolatile printed memory devices have great potential in modern electronic systems such as radio frequency identification tags, portable personal computers and sensors [10] , [11] , [12] , [13] , [14] , [15] , [16] , [17] , [18] , [19] , [20] , [21] . IR-sensing memory array can be used in various applications such as an integrated imaging system or light-assisted special storage; meanwhile, the non-visible light is more suitable for data encryption [22] , [23] . In general, flash memories are programmed, erased and read by applying a voltage bias. There is always a problem of storing confidential information in a flash memory device since the data can easily be retrieved by applying a simple voltage bias. If the device is light driven with a particular narrow width of wavelength in addition to the voltage bias, the stored data could be kept more secure. In this regard, we designed a photonic flash memory device where IR light is used for data encryption in addition to an applied voltage bias. In flash memory device architecture, most of the organic or inorganic semiconductors have almost no absorption in the IR region due to their typical optical energy band gap [24] , [25] , [26] , [27] , [28] . Upconversion (UC) describes a nonlinear optical process, in which a UC material generates one high-energy photon for every two or more low-energy excitation photons. It has been proved to utilize UC materials for optical manipulation in applications such as solid-state lasers, solar energy conversion, optical storage, cancer therapy and biological labelling/imaging [29] , [30] , [31] , [32] , [33] , [34] . UC materials have not been used for flash memories. By the absorption of IR light, high-energy photons are emitted by the UC materials. Eventually, the high-energy emission from UC materials are reabsorbed by the active semiconductor layer and more photoexcitons are generated in the active layer, which ultimately influence the charge-trapping efficiency and data storage levels of the memory device. Nanocrystals dispersed in the semiconductor polymer matrix as the charge-trapping element is a critical step in the quest to fabricate low-cost flash memory [35] , [36] , [37] , [38] . Meanwhile, using nanocrystals as charge-trapping elements can control the trapping levels and sites through solution process, which is highly desirable for printed electronics [39] , [40] , [41] . Finally, with UC nanocrystals dispersed in a three-dimensional space of the polymer matrix, we demonstrate an approach to manipulate the data storage levels with IR assistance. In this article, we have developed a novel photonic flash memory combining multilevel data storage and tunability. Wide-band gap UC materials are used as nanolamps whose visible emission enhances the data storage levels of nonvolatile flash memory. Near-IR light is used to manipulate the stored charges in the flash memory for the multilevel data storage. The active layer materials are nanocomposites composed of Er 3+ , Yb 3+ codoped sodium yttrium fluoride (NaYF 4 ) nanocrystals, which is one of the most promising and effective IR-to-visible UC materials [42] blended with poly(3-hexylthiophene) (P3HT) semiconducting polymer. Undoped NaYF 4 shell is deposited on the surface of NaYF 4 :Yb,Er nanoparticles to enhance the emission intensity. By doping various concentrations of NaYF 4 :Yb/Er@NaYF 4 core–shell nanocrystals in P3HT, we demonstrate tunable photonic memory characteristics with good endurance property, long retention time and multilevel data storage capability. Furthermore, an ultrathin polyethylene naphthalate (PEN)-based flexible photonic memory array has been fabricated to present its compatibility with low voltage operation and high mechanical flexibility. To demonstrate the photonic memory array for practical use, memory array was tested under various bending conditions and found to exhibit stable memory characteristics. Our results demonstrate a novel architecture for photonic nonvolatile flash memory. Device structure Schematic illustration on the working mechanism of the hybrid memory is shown in Fig. 1a . Note that the thickness of each layer is not drawn to scale. Silicon wafer or PEN sheet were used as substrates, and the memory arrays were fabricated on SiO 2 or Al 2 O 3 gate dielectric layers. All the fabricating procedures are compatible with common semiconductor fabrication technology, and the functional device elements (UC nanocrystals/polymer nanocomposites) are suitable for roll-to-roll printing. The UC nanocrystals are the charge-trapping sites in the semiconductor polymer matrix. Under excitation by IR light, the nanocrystals emit photons that are reabsorbed by the polymer. When the photon energy is equal or higher than that of the band gap of the semiconductor polymer, the excitons are generated. A bias at the gate separates the excitons into free electrons and holes. Therefore, more positive-charge carriers are immobilized at the trapping sites under the electrical field ultimately enhancing the programming efficiency due to the IR light. The transmission electron microscope (TEM) image of the NaYF 4 :Yb,Er/NaYF 4 core/shell nanocrystals is shown in Fig. 1b , revealing uniform nanoparticles with diameter of ~30 nm. TEM image of NaYF 4 :Yb,Er nanocrystals without the shell is shown in Supplementary Fig. 1 . Comparison with the core indicates the thickness of the NaYF 4 shell is ~3 nm, which provides an effective barrier to interactions with high-phonon energy environments and shield the core from non-radiative relaxation processes [43] . The oleate-caped nanocrystals are well dispersed in the polymer and form the nanocomposite solution. The core/shell nanocrystals have an absorption peak at 980 nm as shown in Fig. 1c . The absorption spectrum of P3HT in Fig. 1d shows two intrachain π–π* absorption peaks at 520 and 550 nm, and an interchain low-energy shoulder at 600 nm, indicating the crystalline π-stacking structure of P3HT [44] . The photoluminescence (PL) spectrum of the core/shell nanocrystals under excitation wavelength of 980 nm are also illustrated in Fig. 1d . The green emission is attributed to the transitions 2 H 11/2 → 4 I 15/2 and 4 S 3/2 → 4 I 15/2 of Er 3+ ions while the blue emission corresponds to the 2 H 9/2 → 4 I 15/2 transition and the red emission corresponds to the 4 F 9/2 → 4 I 15/2 transition [45] . The nanocrystals in the presence of P3HT have decreased intensity of blue and green emission as shown in Fig. 1e , which indicates that these emissions are successfully reabsorbed by the P3HT molecule through radiative transfer [46] . 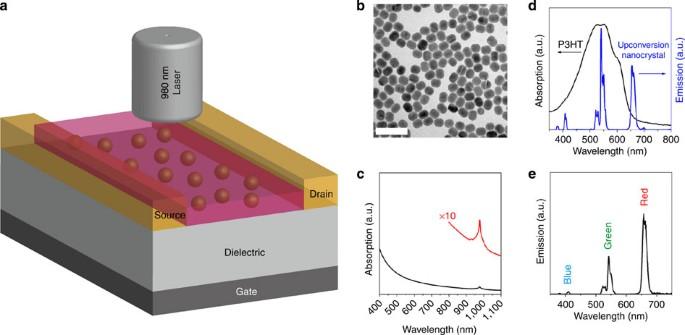Figure 1: Photonic flash memory cell. (a) Illustration of the memory device. (b) TEM image of the core/shell nanocrystals. (c) Absorption spectrum of the core/shell nanocrystals. (d) Absorption spectrum of the P3HT film and photoluminescence spectrum of the core/shell nanocrystals. (e) Photoluminescence spectrum of the core/shell nanocrystals inside the P3HT film. Scale bar, 100 nm (b). Figure 1: Photonic flash memory cell. ( a ) Illustration of the memory device. ( b ) TEM image of the core/shell nanocrystals. ( c ) Absorption spectrum of the core/shell nanocrystals. ( d ) Absorption spectrum of the P3HT film and photoluminescence spectrum of the core/shell nanocrystals. ( e ) Photoluminescence spectrum of the core/shell nanocrystals inside the P3HT film. Scale bar, 100 nm ( b ). Full size image Working mechanism The UC process is illustrated using the energy level diagram shown in Fig. 2a , where the near-IR photons are absorbed by the Yb 3+ ions followed by subsequent energy transfer to Er 3+ ions nearby. The emission peaks of the UC nanocrystals are well matched with the absorption range of P3HT. The sharp emission bandwidths and long excited-state lifetimes of NaYF 4 :Yb/Er@NaYF 4 core–shell nanocrystals are beneficial for the exciton creation in P3HT under IR light. Here, P3HT behaves as an efficient luminescence quencher for the nearby nanocrystals. We further performed time-resolved dynamic studies of the core/shell nanocrystals in the P3HT film. 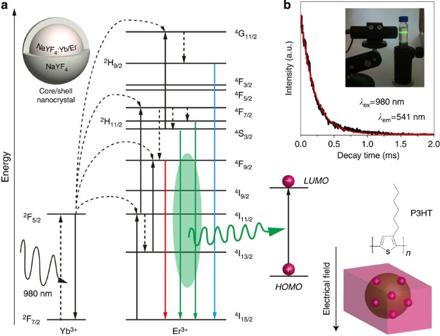Figure 2: Working mechanisms of the nanocomposite system. (a) Energy level and the working mechanism. (b) Luminescence decay curves of the nanocrystals in P3HT film. Inset: the core/shell nanocrystal solution under the illumination of 980 nm laser. Figure 2b shows the luminescence decay curves of the composite film doped with core/shell nanocrystals (1 mg ml −1 ). The curve is well-fitted into a single-exponential function as I = I 0 exp (− t / τ ), where I 0 is the initial emission intensity at t =0 and τ is the lifetime of the Er 3+ ion. The PL lifetime is determined to be ~0.2 ms. The inset shows the image of UC nanocrystals (in cyclohexane) under 980 nm excitation, in which the green emission is consistent with the emission spectrum. The composite with various concentrations of UC nanocrystals show similar decay time ( Supplementary Fig. 2 ), indicating the radiative energy transfer takes place predominately [43] . Figure 2: Working mechanisms of the nanocomposite system. ( a ) Energy level and the working mechanism. ( b ) Luminescence decay curves of the nanocrystals in P3HT film. Inset: the core/shell nanocrystal solution under the illumination of 980 nm laser. Full size image Nanocomposite film The atomic force microscopy topography images of P3HT films doped with nanocrystals are shown in Fig. 3a . Various amounts of NaYF 4 :Yb/Er nanocrystals (in cyclohexane) were mixed with P3HT (in 1,2-dichlorobenzene) and then spin-coated on the substrate. Exact processing details can be found in the Methods section. The root mean square (r.m.s.) surface roughness is summarized in Fig. 3b , and it increases with the doping concentration. The nanocomposite films have also been examined by grazing incidence X-ray diffraction as shown in Fig. 3c . An increase in the doping concentration leads to decreased intensity of (100) peak of P3HT [47] . The (010) peak of P3HT cannot be observed in the pristine P3HT film as well as in nanocomposite films, therefore edge-on orientation of P3HT with respect to the substrate dominates in the composite films, which is favourable for hole transport [48] , [49] . Another diffraction peak in the spectra can be indexed to the hexagonal phase of NaYF 4 , which is regarded as the most effective host matrix for UC fluorescence. The intensity of (100) peak of the nanocrystals increases with its doping amounts, proving that more and more nanocrystals are introduced into the P3HT matrix. As shown in Supplementary Fig. 3 , the ultraviolet–visible spectra of the nanocomposites indicate that the increased doping concentration led to decreased intensity of the absorption peaks, which is consistent with inferior crystallinity of P3HT as evidenced by the X-ray diffraction patterns. Doping the nanocrystals into the P3HT matrix might disturb the lamellar packing of P3HT chains along the crystallographic direction perpendicular to the backbone [50] , therefore the doping concentration is well controlled without sacrificing the device performance. 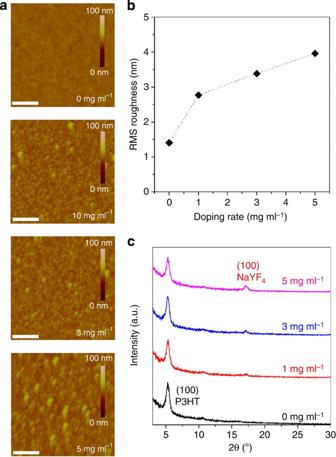Figure 3: Characterization of the nanocomposite films. (a) Atomic force microscopy images of nanocomposite films doped with various amounts of core/shell nanocrystals. (b) Surface roughness of the nanocomposite films with respect to the doping concentration. (c) X-ray diffraction patterns of the nanocomposite films with various concentrations of core/shell nanocrystals in the polymer matrix. Scale bars, 500 nm (a). Figure 3: Characterization of the nanocomposite films. ( a ) Atomic force microscopy images of nanocomposite films doped with various amounts of core/shell nanocrystals. ( b ) Surface roughness of the nanocomposite films with respect to the doping concentration. ( c ) X-ray diffraction patterns of the nanocomposite films with various concentrations of core/shell nanocrystals in the polymer matrix. Scale bars, 500 nm ( a ). Full size image Electrical performance We fabricated hybrid memory transistors both on rigid (100 nm oxide on a heavily doped n-type Si wafer) and flexible polymer substrates. Bottom-gate bottom-contact device structure is used in our study. First, we discuss devices fabricated on rigid Si substrates. The current–voltage characteristics of the memory devices doped with various amount of nanocrystals in P3HT are shown in Fig. 4a–c . It should be noted that all transfer characteristics were measured in a dark environment. For the devices on Si substrates, the OFF state (programmed state) was obtained by applying a gate bias of −40 V for 1 s, and the ON state (erased state) was obtained by applying a gate bias of +40 V for 1 s. The schematic illustrations of the programmed/erased states of the memory device are depicted in Supplementary Fig. 4 . In an OFF device, finite charges are stored at the interface of the UC nanocrystals and polymer, whereas an ON device is referred to a memory state after the stored charges are removed. In the programming process, the holes are transferred and trapped into the nanocrystals and/or interfaces between P3HT and nanocrystals. The stored charge carriers in the nanocrystals provide a built-in potential across the channel and reduce the effective electrical field, leading to a shift in threshold voltage of the two states. The shifts in the threshold voltage were reproducible and fully reversible. In the erasing process, the trapped charge carriers are released. With this program/erase voltage, the pristine P3HT devices had almost no charging effects, and they showed negligible shifts in the transfer curves with a hole mobility of ~0.05 cm 2 V −1 s −1 ( Supplementary Fig. 5 ). The memory window (the threshold voltage shifts) increases from 1.9 to 7.4 V (~6.3% to ~24.7% of the working voltage) when the doping concentration of UC nanocrystals increase from 1 to 5 mg ml −1 as shown in Fig. 4d . Meanwhile, the mobilities of the nanocomposite film are found to decrease as the doping concentration increases, suggesting that the charge transport is affected by the addition of nanocrystals. A further increase in doping concentration will lead to degradation in device performance. Therefore, we chose an optimum doping concentration of 5 mg ml −1 to study the photonic memory behaviour. During the programming process, the devices were illuminated by 200 mW 980 nm laser. The transfer curves of ON and OFF states are shown in Fig. 4e . The output characteristics of the memory device in ON and OFF states are shown in Supplementary Figs 6 and 7 , respectively. The memory window increased to 10.2 V (~34% of the working voltage) with IR assistance, demonstrating more charge carriers are trapped in the nanocrystals. Under the illumination of 980 nm laser, the UC nanocrystals emit green light, which is simultaneously reabsorbed by P3HT. The photoinduced electron–hole pairs are separated with the application of a negative gate bias, and more holes are trapped in the nanocrystals during the programming process under IR illumination ( Supplementary Fig. 4 ). The IR tunable memory effect can be applied in a multilevel memory cell, in which more than one single bit can be stored ( Supplementary Fig. 8 ). The different states of the memory cell are attributed to the different degrees of trapping with and without IR illumination. The difference between the two states also demonstrates the use of IR for the photonic memory encryption.Unlike dynamic random access memory, nonvolatile memory retains the information when the power is turned off [51] . The data retention property of the multilevel IR laser-assisted hybrid memory is shown in Fig. 4f . The reading bias at gate and drain were set as 5 V and −5 V, respectively. After 10 5 s, the hybrid memory cell still exhibited well-separated data states, demonstrating the holes were confined well in the core/shell nanocrystals. Possible charge loss may occur in the nanocomposite film from the nanocrystals to active channel. However, the degradation of retention properties of our memory device is not severe due to the long-chain organic ligand covering the nanocrystals and the large band gap NaYF 4 shell, which can form an insulating barrier to prevent the diffusion of the trapped charge carriers [52] . 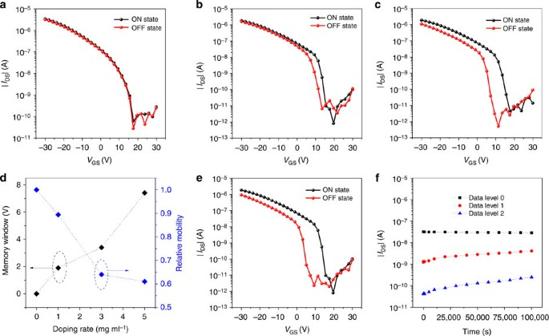Figure 4: Memory characteristics of the hybrid memory. (a) Transfer curves of the memory device doped with 1 mg ml−1core/shell nanocrystals. (b) Transfer curves of the memory device doped with 3 mg ml−1core/shell nanocrystals. (c) Transfer curves of the memory device doped with 5 mg ml−1core/shell nanocrystals. (d) Memory windows and relative mobilities as a function of doping concentration. (e) Memory characteristics of the memory device with IR-assisted programming behaviour. (f) Retention property of the multilevel IR photonic memory device. Figure 4: Memory characteristics of the hybrid memory. ( a ) Transfer curves of the memory device doped with 1 mg ml −1 core/shell nanocrystals. ( b ) Transfer curves of the memory device doped with 3 mg ml −1 core/shell nanocrystals. ( c ) Transfer curves of the memory device doped with 5 mg ml −1 core/shell nanocrystals. ( d ) Memory windows and relative mobilities as a function of doping concentration. ( e ) Memory characteristics of the memory device with IR-assisted programming behaviour. ( f ) Retention property of the multilevel IR photonic memory device. Full size image Ultra flexible device We further demonstrate the hybrid memory on flexible PEN substrate. Until now, there are very few reports of hybrid flash memory devices, most of which use rigid substrate [53] , [54] or large program/erase voltage [55] . Here we use the atomic layer deposition method to fabricate the aluminium oxide (Al 2 O 3 ) dielectric layer at low temperature, demonstrating good reproducibility and sufficient uniformity with high device yields. The program and erase voltage is reduced as low as −5 V and +5 V for 1 s, respectively. 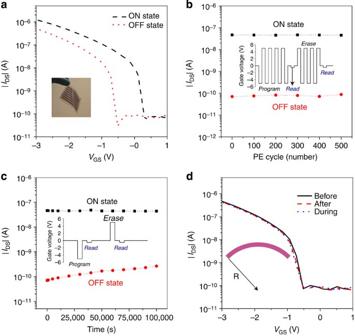Figure 5: Ultra flexible photonic memory device. (a) Transfer characteristics of the IR photonic memory device with low voltage operation. Inset: optical image of the flexible memory array on a PEN film. (b) Endurance characteristics of the memory device as a function of program/erase cycles. Inset: test pulse sequence for the endurance test. (c) Data retention property of the memory device. Inset: test pulse sequence for the retention test. (d) Transfer curves of the flexible memory device before, during and after the bending test. Inset: illustration of the memory cell under bending test. Figure 5a shows the transfer curves of the ON and OFF states under IR illumination. The inset shows a photograph of a 12-μm-thin PEN plastic sheet that consists of an array of memory transistors. The operation of flexible memory under dark conditions is shown in Supplementary Fig. 9 . In the reading process, the bias at gate and drain were both set as −0.5 V. The flexible device works well under −3 V and the reading ON/OFF current ratio is around 10 3 . The memory window is found to be 30% of the working voltage and sufficient for reliable memory operation under IR illumination. Program/erase cycling test was carried out and the results are depicted in Fig. 5b . The test pulse sequence for the endurance measurement is shown in the inset. Over 500 repeated programming and erasing cycles have been demonstrated at room temperature without degradation. A number of program/erase cycles over several hundreds were believed to be promising for applications in low-cost and low-power flexible electronics [56] , [57] . The data retention properties were measured as a function of time at room temperature. The ON and OFF currents were well separated with respect to the elapsed time as shown in Fig. 5c , which is comparable to other reported values [13] , [58] . The inset shows the test pulse sequence for the data retention measurement. The bending stability is an important factor for flexible electronic devices [59] . The hybrid memory device exhibits almost no change in the OFF state before and after bending the flexible substrate as shown in Fig. 5d . The substrate with memory array was bent with a radius of curvature of 5 mm, which leads to a tensile strain of −0.12% (ref. 60 ). The memory properties were well maintained during the bending test, confirming the nanocrystal/P3HT composite layer is suitable for flexible electronics. Figure 5: Ultra flexible photonic memory device. ( a ) Transfer characteristics of the IR photonic memory device with low voltage operation. Inset: optical image of the flexible memory array on a PEN film. ( b ) Endurance characteristics of the memory device as a function of program/erase cycles. Inset: test pulse sequence for the endurance test. ( c ) Data retention property of the memory device. Inset: test pulse sequence for the retention test. ( d ) Transfer curves of the flexible memory device before, during and after the bending test. Inset: illustration of the memory cell under bending test. Full size image We have demonstrated a photonic nonvolatile memory device with hybrid polymer/UC nanocrystal composite as an active layer. By controlling the doping concentration of nanocrystals, the memory properties have been systematically tuned. The advantage of our approach is that the memory density can be increased in a three-dimensional space of the polymer matrix, which is instrumental in miniaturization of flexible flash memory. With the assistance of IR, we obtained a multilevel memory cell in which more than one single bit could be stored. In addition, we demonstrate an IR flash memory that can also be extended to other application such as IR sensing. Our approach opens a way for future design of photonic wearable memory devices that could be programmed/erased with IR light. Materials P3HT (regioregular), Yttrium(III) acetate hydrate (99.9%), ytterbium(III) acetate hydrate (99.9%), erbium(III) acetate hydrate (99.9%), sodium hydroxide (NaOH, >98%), ammonium fluoride (NH 4 F, >98%), 1-octadecene (90%) and oleic acid (90%) were purchased from Sigma-Aldrich. All the starting materials and solvents were used without further purification. The PEN substrates were provided by DuPont Teijin Films China Limited. Synthesis of the UC nanoscrystals The nanoparticles synthesis developed via a modified wet chemical procedure [61] . In a typical procedure to the synthesis of NaYF 4 :Yb/Er nanoparticles, 2-ml water solution of Ln(CH 3 CO 2 ) 3 (0.2 M, Ln=Y, Yb and Er) was added to a 50-ml flask containing 3 ml of oleic acid and 7 ml of 1-octadecene. The mixture was heated at 160 °C for 40 min to form the lanthanide–oleate complexes and then cooled down to 50 °C naturally. Thereafter, 5 ml of methanol solution containing NH 4 F (1.6 mmol) and NaOH (1 mmol) was added and the resultant solution was stirred for 30 min. After the methanol was evaporated, the solution was heated to 290 °C under argon for 1 h and then cooled down to room temperature. The resulting nanoparticles were precipitated by the addition of ethanol, collected by centrifugation at 6,000 r.p.m. for 5 min, washed with ethanol several times and re-dispersed in 4 ml of cyclohexane. The core–shell nanoparticles were synthesized by a similar procedure, except that preformed core nanoparticles dispersed in cyclohexane were added along with a methanol solution of NH 4 F and NaOH to initiate an epitaxial shell growth process. Device fabrication For the rigid device, the silicon wafer with 100 nm SiO 2 was used as the substrate. The wafers were cleaned in deionized water, acetone and iso-propanol for 15 min (each) using an ultrasonic bath and dried with nitrogen gas before use. The 50-nm Au source and drain contacts were deposited on the SiO 2 with a channel length (L) to width (W) ratio as 6 μm to 3,000 μm. P3HT was dissolved in 1,2-dichlorobenzene, and then blended with different concentrations of NaYF 4 :Yb/Er nanoparticles. Ultrasonification was carried out for 30 min to further promote a stable dispersion of nanocrystals. No apparent precipitation was found for all the concentration of nanocomposite solutions. The mixed nanocomposite solutions and pure P3HT solution were spin-coated on the as-fabricated substrates followed by 130 °C annealing for 20 min in the nitrogen glove box, resulting in a thickness of ~30 nm for the film. Flexible memory devices were fabricated on a 12-μm-thick PEN film. Two hundred-micrometer-thick polyethylene terephthalate sheets were used as supporting substrates to ease handling of the PEN substrate during the device fabrication process. A 30-nm Ag was deposited as the gate electrode through a shadow mask at a pressure of 3 × 10 −6 mbar and a rate of 0.02 nm s −1 . A 15-nm Al 2 O 3 layer was deposited as a gate dielectric using a Savannah 100 ALD system at a substrate temperature of 80 °C. A 50-nm Au source and drain contacts were deposited on the Al 2 O 3 with a channel length (L) to width (W) ratio as 30 μm to 1,000 μm for a single transistor. The other processes are the same as rigid devices. Characterization The size distribution of the UC nanocrystals was verified by TEM (Philips CM20). The thicknesses of the deposited layers were measured using the ellipsometer. The morphologies of these films were investigated by atomic force microscope (Veeco Multimode V). Grazing incidence X-ray diffraction pattern of the films were recorded using an X-ray diffractometer (Rigaku SmartLab). Irradiation of parallel CuK α1,2 X-ray beam was fixed at a grazing incident angle of 0.5°, and the detector was independently moved to collect the diffraction data with a step-size of 0.02°. The absorption spectrum was obtained using a SHIMADZU UV-1700 spectrophotometer. The steady-state PL spectra were recorded at room temperature with an F-4600 spectrophotometer (Hitachi) with the excitation source adapted to fibre-coupled diode lasers. PL decay curves were measured on an Edinburgh FLS920P spectrometer equipped with a 980-nm diode laser that is modulated to provide the excitation pulses. The bending experiments were achieved by bending the flexible PEN substrates on selected convex radii. The electrical characteristics of the transistors were measured using a Keithley 2612 source meter at room temperature in a nitrogen glove box. How to cite this article: Zhou, Y. et al. An upconverted photonic nonvolatile memory. Nat. Commun. 5:4720 doi: 10.1038/ncomms5720 (2014).